Environmental impact on direct neuronal reprogrammingin vivoin the adult brain Direct reprogramming of non-neuronal cells to generate new neurons is a promising approach to repair damaged brains. Impact of the in vivo environment on neuronal reprogramming, however, is poorly understood. Here we show that regional differences and injury conditions have significant influence on the efficacy of reprogramming and subsequent survival of the newly generated neurons in the adult rodent brain. A combination of local exposure to growth factors and retrovirus-mediated overexpression of the neurogenic transcription factor Neurogenin2 can induce new neurons from non-neuronal cells in the adult neocortex and striatum where neuronal turnover is otherwise very limited. These two regions respond to growth factors and Neurogenin2 differently and instruct new neurons to exhibit distinct molecular phenotypes. Moreover, ischaemic insult differentially affects differentiation of new neurons in these regions. These results demonstrate strong environmental impact on direct neuronal reprogramming in vivo . The discovery of induced pluripotent stem cells has transformed our view on the cell-type specificity in the animal body [1] . Combinatorial overexpression of just a few regulatory molecules can covert fully differentiated cells into most primitive pluripotent stem cells, demonstrating that cell-type specification is reversible and reprogrammable [1] , [2] . Recent studies have further demonstrated that fully functional mature cells with particular cell types such as neurons and cardiac muscle cells can be directly generated in vitro from other cell types without passing through the stage of induced pluripotent stem cells [3] . Generation of tissue-specific stem/progenitor cells such as neural stem cells from fibroblasts has also been reported [3] . This direct reprogramming is a promising approach to obtain new functional cells and replace those lost to insults, the ultimate goal in regenerative medicine [2] , [3] . Most studies so far reported, however, have utilized in vitro culture to convert one cell type to the other, and some studies [4] , [5] , [6] , [7] , [8] , [9] , [10] have shown that direct reprogramming is also possible in vivo in adult organs, including the brain [8] , [9] , [10] . Yet, little is known thus far about the environmental influences on such in vivo reprogramming events. Cell reprogramming involves extensive epigenetic modifications [2] , [3] , and therefore, the complex in vivo environment is likely to have substantial influences on the process. Currently, little is known about the environmental impact on direct reprogramming. In the adult mammalian brain, neurogenesis persists only in a few restricted regions, including the subventricular zone (SVZ) lining the lateral ventricle and the hippocampal dentate gyrus [11] . In these so-called neurogenic regions, adult neural stem/progenitor cells (herein collectively called NPCs) serve as the source of new neurons [11] . Whether the production of new neurons also occurs in other regions of the intact brain remains controversial [12] , [13] . Nevertheless, recent studies have demonstrated that various insults induce new neurons in normally non-neurogenic regions [14] , [15] , [16] . These newly generated neurons in the injury site, however, are relatively small in number and survive only for a short period [15] , [16] . Given such a limited regenerative capacity, approaches alternative to the mobilization of endogenous NPCs need to be pursued, and cell reprogramming is one of such promising strategies. In this study, we show that a combination of growth factors (GFs) and the neurogenic transcription factor (TF) Neurogenin2 (Neurog2) [17] induces new neurons from non-neuronal cells in situ in the adult rodent neocortex and striatum where neuronal turnover is otherwise restricted. We found that these two brain regions respond to GFs and Neurog2 differently and instruct new neurons to exhibit distinct phenotypes. Moreover, ischaemic insult differentially modulates differentiation of new neurons in these regions. These results highlight strong environmental impact on direct neuronal reprogramming in vivo . In vivo manipulations using GFs and retroviruses Previous studies have demonstrated that a combination of a few TFs can directly convert non-neuronal cells to functional neurons [18] , [19] , [20] , [21] , [22] , [23] , [24] , [25] , [26] . Although much attention has been focused on how these TFs modify the epigenetic landscape of target cells, an often-ignored condition is that reprogrammed cells are exposed to various growth stimuli and undergo multiple cell divisions in culture. Thus, we sought to test whether an exposure to a high-dose GF augments cell reprogramming in vivo . As a means to genetically manipulate cells, we took advantage of the fact that retroviruses selectively infect proliferative cells, but not postmitotic neurons. To minimize false labelling of postmitotic cells and cell fusion between virus-infected cells and pre-existing neurons [27] , we used the non-pseudotyped vector pMXIG expressing enhanced green fluorescent protein (GFP) [9] , [17] . We created stab wound at defined locations in the striatum and neocortex of the adult rat brain by focal injection of high-titer viruses, with or without a cocktail of fibroblast growth factor 2 (FGF2) and epidermal growth factor (EGF). Target areas were chosen to avoid labelling of endogenous NPCs and their progeny in the nearby SVZ and rostral migratory stream ( Fig. 1a–c ). In fact, virus-infected cells were found as a cluster of GFP + cells confined to the area around the injected site at day 3 after infection (DAI-3; Fig. 1d–k ), and pre-labelling of NPCs with 5-bromo-2′-deoxyuridine (BrdU) before virus infection yielded few, if any, GFP/BrdU-double-labelled cells in the SVZ or RSM ( Supplementary Fig. S1 ). A subset of GFP-labelled cells expressed glial fibrillary acidic protein (GFAP), NG2, nestin and Olig2, known markers for NPCs and glial progenitors ( Supplementary Fig. S2 ). We also identified RECA1 + vascular endothelial cells and OX42 + microglia/macrophages among GFP + cells. These populations, as a whole, however, comprised <50% of the total labelled cells. Importantly, no GFP + cells co-expressed neuronal markers in either the striatum or neocortex at DAI-3 (none among over 3,000 cells examined in each region). Thus, labelling of pre-existing neurons by GFP viruses was, if any occurred, below the detectable level. Even at later time points, few cells infected with control viruses alone expressed neuronal markers (2 GFP + /NeuN + cells out of 5,112 cells in the striatum and none out of 4,258 cells in the neocortex at DAI-14). These results are consistent with previous studies reporting limited neurogenesis after stab injury [28] , [29] . 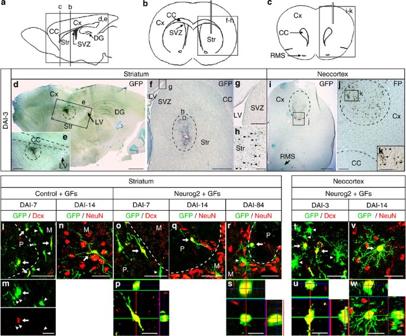Figure 1: Focal labelling of striatal and neocortical cells with GFP retroviruses in the adult rat brain. (a–c) Schematic diagrams illustrating the location of virus injection sites in parasagittal (a) and coronal (b,c) views. Boxes ina,b, andcindicate the areas shown ind,f, andj, respectively. (d–k) Distributions of GFP+cells (dashed circles and arrowheads) in the striatum (d–h) and neocortex (i–k) at DAI-3. Sections were counterstained with methylgreen. Boxes ind,f, andjindicate the areas shown ine,gandh,j, andk, respectively. (l–w) Co-expression of neuronal markers and GFP in virus-infected cells (arrows) in the striatum (l–s) and neocortex (t–w). Dashed lines inl,o,q,rindicate the border of the matrix (M) and patch (P) compartments of the striatum. Arrows and arrowheads indicate GFP+cells co-expressing and non-expressing, respectively, the marker shown above each panel. The lower panelsm,p,s,u,wshow the colocalization of relevant markers in single cells in orthogonal views of confocal z-stack images ini,o,r,t,v, respectively. Scale bar,d,e,f,i, 1 mm;e,g,h,j,k, 100 μm;l,n,o,q,r,t,v, 50 μm;m,p,s,u,w, 20 μm. Cx, neocortex; CC, corpus callosum; DG, dentate gyrus; LV, lateral ventricle; RMS, rostral migratory stream; Str, striatum; SVZ, subventricular zone. Figure 1: Focal labelling of striatal and neocortical cells with GFP retroviruses in the adult rat brain. ( a – c ) Schematic diagrams illustrating the location of virus injection sites in parasagittal ( a ) and coronal ( b , c ) views. Boxes in a , b , and c indicate the areas shown in d , f , and j , respectively. ( d – k ) Distributions of GFP + cells (dashed circles and arrowheads) in the striatum ( d – h ) and neocortex ( i – k ) at DAI-3. Sections were counterstained with methylgreen. Boxes in d , f , and j indicate the areas shown in e , g and h , j , and k , respectively. ( l – w ) Co-expression of neuronal markers and GFP in virus-infected cells (arrows) in the striatum ( l – s ) and neocortex ( t – w ). Dashed lines in l , o , q , r indicate the border of the matrix (M) and patch (P) compartments of the striatum. Arrows and arrowheads indicate GFP + cells co-expressing and non-expressing, respectively, the marker shown above each panel. The lower panels m , p , s , u,w show the colocalization of relevant markers in single cells in orthogonal views of confocal z-stack images in i , o , r , t , v , respectively. Scale bar, d , e , f , i , 1 mm; e , g , h , j , k , 100 μm; l , n , o , q , r , t , v , 50 μm; m , p , s , u , w , 20 μm. Cx, neocortex; CC, corpus callosum; DG, dentate gyrus; LV, lateral ventricle; RMS, rostral migratory stream; Str, striatum; SVZ, subventricular zone. Full size image GFs and Neurog2 promote neuronal reprogramming in vivo We then asked whether GFs and Neurog2 promote neurogenesis. We observed no significant change in the spectrum of cell types among virus-infected cells in GF-treated animals, and few GFP + cells were Dcx + or NeuN + at DAI-3. Nonetheless, a small fraction of GFP + cells expressing Dcx and NeuN were detected at DAI-7 and DAI-14, respectively, in the striatum ( Fig. 1l–m ). No such cells were detected, however, in the GF-treated neocortex. Given this limited action of GFs, we next used Neurog2 viruses. In the striatum, Neurog2 viruses alone and Neurog2 together with GFs significantly increased GFP + /Dcx + and GFP + /NeuN + cells ( Fig. 1o–s ; for quantification, see Fig. 2 ). Neuronal differentiation of GFP + cells was also demonstrated by co-labelling with β-tubulin type III (TuJ1), MAP2 and HuC/D ( Fig. 4a–e ). Approximately three-fourth of these neuronal marker-positive GFP + cells (72±5%, n =3 animals) were Neurog2 + at DAI-7, but a much small fraction (17±4%) retained Neurog2 expression at DAI-28 or later despite the sustained GFP expression, suggesting that the transgene is silenced over time. 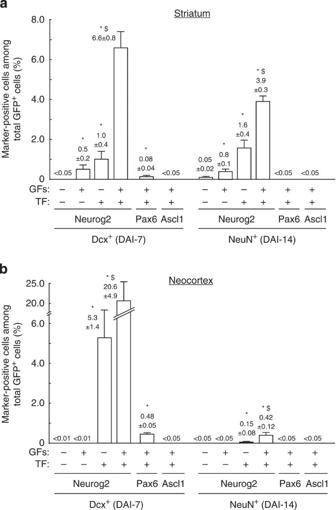Figure 2: Differential impacts of GFs and Neurog2 in neuronal induction in the adult rat striatum and neocortex. The percentages of GFP+cells expressing Dcx and NeuN in the striatum (a) and neocortex (b) under various conditions are shown (mean±s.d.,n=3–4 animals). GFP+/Dcx+cells were examined at DAI-3 and DAI-7 in the neocortex and striatum, respectively. *P<0.01 compared with control viruses in Student’st-test; $P<0.01 compared with treatment with GFs or Neurog2 viruses alone in Student’st-test. Figure 2: Differential impacts of GFs and Neurog2 in neuronal induction in the adult rat striatum and neocortex. The percentages of GFP + cells expressing Dcx and NeuN in the striatum ( a ) and neocortex ( b ) under various conditions are shown (mean±s.d., n =3–4 animals). GFP + /Dcx + cells were examined at DAI-3 and DAI-7 in the neocortex and striatum, respectively. * P <0.01 compared with control viruses in Student’s t -test; $ P <0.01 compared with treatment with GFs or Neurog2 viruses alone in Student’s t -test. Full size image Figure 4: Region-specific differentiation of GFP-labelled neurons in the striatum and neocortex. 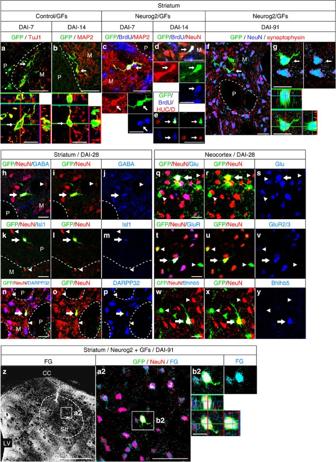Figure 4: Region-specific differentiation of GFP-labelled neurons in the striatum and neocortex. (a–g) Co-labelling of various neuronal markers and BrdU in GFP+cells (arrows) in the striatum. Time points after infection, types of manipulations used and markers stained are shown above individual panels. Inc–e, BrdU was administered twice each day for 3 days between DAI-0 and DAI-2. Dashed lines ina-c,findicate the border of the matrix (M) and patch (P) compartments of the striatum. Lower panels ina–d,gshow orthogonal views of confocal z-stack images of the cells indicated by arrows. Note that the overlap of green, red and blue colours inc–eis indicated as white colour. (h–y) Region-specific phenotypes of GFP-labelled neurons in the striatum (h–p) and neocortex (q–y) at DAI-28. Arrows indicate GFP+/NeuN+neurons expressing relevant markers, whereas arrowheads indicate marker-negative GFP+and/or NeuN+cells. Images inn–pwere obtained from control virus-infected animals, whereas all others were from Neurog2 virus-infected animals. (z,b2) Retrograde labelling of GFP+/NeuN+cells in the striatum by FG. FG was injected into the globus pallidus ipsilateral to the virus injection site at DAI-84, and animals were analysed at DAI-91.zshows the distribution of FG fluorescence (white dots) in the striatum (the virus injection site in a dashed circle).a2shows GFP+/NeuN+cells co-labelled with FG detected in the area boxed inz.b2shows confocal images (an orthogonal view in lower panels) of a neuron boxed ina2. Scale bar,a–g, 50 μm;h–y, 25 μm;z, 1 mm;a2, 50 μm;b2and lower panels ofa-d,gandb2, 20 μm. ( a – g ) Co-labelling of various neuronal markers and BrdU in GFP + cells (arrows) in the striatum. Time points after infection, types of manipulations used and markers stained are shown above individual panels. In c – e , BrdU was administered twice each day for 3 days between DAI-0 and DAI-2. Dashed lines in a - c , f indicate the border of the matrix (M) and patch (P) compartments of the striatum. Lower panels in a – d , g show orthogonal views of confocal z-stack images of the cells indicated by arrows. Note that the overlap of green, red and blue colours in c – e is indicated as white colour. ( h – y ) Region-specific phenotypes of GFP-labelled neurons in the striatum ( h – p ) and neocortex ( q – y ) at DAI-28. Arrows indicate GFP + /NeuN + neurons expressing relevant markers, whereas arrowheads indicate marker-negative GFP + and/or NeuN + cells. Images in n – p were obtained from control virus-infected animals, whereas all others were from Neurog2 virus-infected animals. ( z , b2 ) Retrograde labelling of GFP + /NeuN + cells in the striatum by FG. FG was injected into the globus pallidus ipsilateral to the virus injection site at DAI-84, and animals were analysed at DAI-91. z shows the distribution of FG fluorescence (white dots) in the striatum (the virus injection site in a dashed circle). a2 shows GFP + /NeuN + cells co-labelled with FG detected in the area boxed in z . b2 shows confocal images (an orthogonal view in lower panels) of a neuron boxed in a2 . Scale bar, a – g , 50 μm; h – y , 25 μm; z , 1 mm; a2 , 50 μm; b2 and lower panels of a - d , g and b2 , 20 μm. Full size image In the neocortex, Neurog2 robustly increased GFP + /Dcx + cells at DAI-3 ( Fig. 1t,u ). Only a small fraction of GFP + cortical cells, however, expressed NeuN at DAI-14 ( Fig. 1v,w ). We tested two other neurogenic TFs, Pax6 and Ascl1. Consistent with a previous report [8] , a small percentage of cells infected with Pax6 viruses became Dcx + in the striatum and neocortex (0.1% and 0.5%, respectively; Fig. 2a,b ). Few GFP + /NeuN + cells, however, were detectable at later time points. Ascl1 did not promote neurogenesis at a detectable level in either regions, in agreement with previous studies [9] , [30] ( Fig. 2a,b ). Ascl1 alone is a potent inducer of neurogenesis in both NPCs [31] and fibroblasts in vitro [18] , [19] , [20] , [21] , [22] , [23] , [24] , [25] , [26] , and can induce new neurons in vivo in combination with other TFs [10] . Thus, its inability to induce new neurons in vivo suggests a significant difference between in vivo and in vitro conditions. We next asked whether GFP + neurons are generated by cells that divide in situ . When BrdU was administered before stab wound, we did not detect any BrdU-labelled neurons around the stab wound ( Supplementary Fig. S1 ). However, when BrdU was administered to animals twice a day for 3 days between DAI-0 and DAI-2, 18±6% of GFP + /MAP2 + cells at DAI-7 and 12±4% of GFP + /NeuN + cells at DAI-14 ( n =3 animals) were co-labelled with BrdU in the Neurog2/GF-treated striatum ( Fig. 4c,d ). BrdU-labelled neurons were also found in Neurog2/GF-treated neocortex at DAI-14 (8±3% of GFP + /NeuN + cells examined, n =3). These results suggest that a significant fraction of GFP-labelled neurons originate from cells that proliferate after injury. Several lines of evidence argue against the idea that GFP-labelled neurons result from infection of pre-existing neurons or cell fusion. First, it has been reported that NeuN + neurons fused with vesicular stomatitis virus coat protein G-pseudotyped retrovirus-infected microglia/macrophages are barely detectable in the adult neocortex [27] . In fact, few cells infected with control viruses co-expressed Dcx or NeuN in our study. Second, such falsely labelled neurons, if ever exist, would emerge within a day after infection and do not survive longer than a week [13] , [27] . In our study, however, a relatively large number of labelled neurons emerged late after infection, and many of them remained weeks after labelling (see below). Finally, the aforementioned BrdU labelling demonstrates that GFP-labelled neurons derive from cells that divide after injury. Together, these data support the idea that GFs and Neurog2 induce new neurons from non-neuronal cells in vivo . Differential actions of GFs and Neurog2 To compare the environmental influence in the striatum and neocortex, we estimated the number of new neurons induced under various conditions based on the quantification of the total number of GFP + cells and the percentage of cells expressing neuronal markers among them at different time points ( Fig. 3a and Supplementary Table S1 ). In the striatum, stab wound alone induced few GFP + /Dcx + or GFP + /NeuN + cells, but GF treatment produced a small but significant number of labelled neurons ( Fig. 3b–d ). Although GFs slightly increased the total number of GFP + cells compared with control (1.2-fold), the net increases in the number of GFP-labelled neurons were much larger (>20-fold), indicating that the effect of GFs is not simply the expansion of virus-infected cells ( Fig. 3d ). Neurog2 stimulated the generation of GFP + /NeuN + cells despite a slight decrease in the number of infected cells ( Fig. 3a,d ). Moreover, the combination of GFs and Neurog2 led to a marked increase of GFP + /Dcx + and GFP + /NeuN + cells, demonstrating their synergistic actions. Importantly, GFP + /Dcx + cells emerged between DAI-3 and DAI-7 but disappeared by DAI-14 ( Fig. 3b ). By contrast, GFP + /NeuN + cells became detectable at DAI-7 onwards and over 60% of those detected at DAI-14 appeared to remain at DAI-84 ( Fig. 3c ). 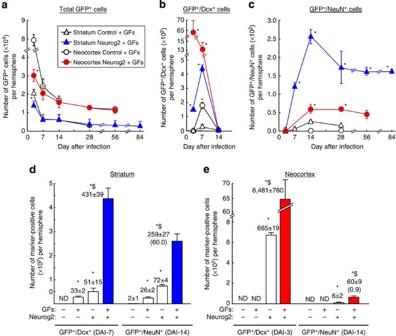These results suggest that new neurons first emerge as Dcx + immature cells and subsequently become NeuN + , reinforcing the idea that GFs and Neurog2 promote the de novo production of neurons, not the survival of falsely labelled pre-existing neurons. Figure 3: Combinatorial actions of GFs and Neurog2. (a–c) The numbers of total GFP+(a), GFP+/Dcx+(b) and GFP+/NeuN+(c) cells detected at different time points after GF/virus infection (mean±s.d.,n=3–4 animals). The number of GFP+cells in GF-untreated animals is shown inSupplementary Table S1. *P<0.01 compared with control viruses in Student’st-test. (d,e) The estimated numbers of GFP+/Dcx+(left) and GFP+/NeuN+(right) cells in the striatum (d) and neocortex (e) under various conditions (mean±s.d.,n=3–4 animals). The numbers in parentheses show the percentage of GFP+/NeuN+cells at DAI-14 compared with GFP+/Dcx+cells at earlier time points. *P<0.01 compared with control viruses in Student’st-test; $P<0.01 compared with GFs or Neurog2 alone in Student’st-test. ND, not detected. Figure 3: Combinatorial actions of GFs and Neurog2. ( a – c ) The numbers of total GFP + ( a ), GFP + /Dcx + ( b ) and GFP + /NeuN + ( c ) cells detected at different time points after GF/virus infection (mean±s.d., n =3–4 animals). The number of GFP + cells in GF-untreated animals is shown in Supplementary Table S1 . * P <0.01 compared with control viruses in Student’s t -test. ( d , e ) The estimated numbers of GFP + /Dcx + (left) and GFP + /NeuN + (right) cells in the striatum ( d ) and neocortex ( e ) under various conditions (mean±s.d., n =3–4 animals). The numbers in parentheses show the percentage of GFP + /NeuN + cells at DAI-14 compared with GFP + /Dcx + cells at earlier time points. * P <0.01 compared with control viruses in Student’s t -test; $ P <0.01 compared with GFs or Neurog2 alone in Student’s t -test. ND, not detected. Full size image Unlike in the striatum, neither stab wound nor GFs alone induced new neurons in the neocortex ( Fig. 3e ). Although Neurog2 induced a large number of GFP + /Dcx + cells at DAI-3, only a few GFP + /NeuN + cells were found at DAI-14 ( Fig. 3b,c,e ). The addition of GFs increased GFP + /Dcx + cells, but again, only a few GFP + /NeuN + cells were found at DAI-28 (0.9% of GFP + /Dcx + cells found at DAI-3; Fig. 3e ). Thus, the actions of GFs and Neurog2 differ in the neocortex and striatum, and the production and/or maturation of new neurons appears more restricted in the neocortex. From the above data, we estimated the extent of neuronal replacement. Stab wound combined with GFs and Neurog2 viruses caused a loss of 3,836±619 and 1,866±129 neurons in the striatum and neocortex, respectively ( n =3 animals). Thus, the estimated replacement rate was 4.6% in the striatum and 3.2% in the neocortex at DAI-28. Although these rates are not remarkable in light of neuronal replacement, they are comparable to those reported for other injury conditions [15] , [16] . Given the fact that GFP viruses infected only a small number of cells in a focal area in our study, the actual potential of neuronal replacement in vivo , if a large number of cells in a widespread region are targeted, could be much greater than this estimation. Region-specific differentiation of new neurons We next examined the molecular phenotypes of newly generated neurons. GFP-labelled striatal neurons were found in both the patch and matrix compartments ( Fig. 4a–c,h–p ) and surrounded by synaptophysin + synaptic speckles similar to neighbouring neurons ( Fig. 4f,g ). Many of them were immunopositive for γ-amino butyric acid (GABA; 76 cells/76 cells examined in three animals) and Isl1 (18 cells/36 cells), reminiscent of differentiating striatal projection neurons ( Fig. 4h–m ). Although Neurog2 drives differentiation programmes of cortical neurons when robustly overexpressed in the developing ventral telencephalon [32] , it also supports the production of striatal neurons when expressed moderately [33] . One exceptional marker was DARPP32. Although many GFP + /NeuN + cells expressed DARPP32 in the control virus-infected striatum (22 cells/50 cells; Fig. 4n–p ), none of the Neurog2 virus-infected cells were DARPP32 + (0/118 cells). Thus, Neurog2 seemed to bias the phenotype of new neurons towards DARPP32 − cells. To examine the connectivity of these neurons, the axonal tracer Fluoro-Gold (FG) was injected into the globus pallidus, one of the targets for striatal neurons at DAI-84. In these animals, punctuated FG labelling surrounded GFP + /NeuN + cells at DAI-91 (8 cells/19 cells examined; Fig. 4z,a2 ). FG labelling was predominantly associated with the soma ( Fig. 4 ), demonstrating that labelling was because of retrograde labelling but not passive diffusion. In the neocortex, few GFP + neurons were found in control virus-infected animals, and therefore we focused on GF/Neurog2-treated animals. We detected GFP + /NeuN + cells immunopositive for glutamate (Glu; 18 cells/18 cells), glutamate receptor subunits 2/3 (GluR2/3; 13 cells/13 cells), and Bhlhb5 (17 cells/29 cells) in multiple layers at DAI-28 ( Fig. 4q–y ). Unlike in the striatum, no GABA + GFP + /NeuN + cells were found in the neocortex. These features resembled those of glutamatergic cortical neurons. Neurog2 viruses and GFs induced GFP-labelled neurons with similar phenotypes in the frontal, parietal and occipital areas ( Supplementary Fig. S3 ). Thus, although induced by the same manipulations, new neurons exhibit distinct molecular phenotypes in different environments. Impact of ischaemia on neuronal induction In the above studies, stab wound was the underlying injury condition. We next examined how ischaemic injury affects neuronal reprogramming. We used a model that produces localized damage in the antero-lateral neocortex, leaving the striatum and other regions largely intact ( Fig. 5a,d,g,k ) [34] . Ischaemia induced expansion of Dcx + neurons in the SVZ beyond its normal boundary with the adjacent striatum [15] , [16] ( Supplementary Fig. S4 ). To distinguish SVZ- and striatal parenchyma-derived neurons, we first labelled SVZ cells with BrdU before ischaemia, and subsequently labelled parenchymal cells with GFP viruses at DAI-0 (see Supplementary Fig. S2a ). Few GFP-labelled neurons were detected in the control virus-infected striatum, indicating that the impact of ischaemia alone was minimum ( Fig. 5o ). Neurog2 viruses and GFs induced a cluster of GFP + /Dcx + and GFP + /NeuN + cells around the injection site, but not near the lateral ventricle (LV) ( Fig. 5b,c,e,f ), and ischaemia modestly increased these cells ( Fig. 5o ). None of these cells were co-labelled with BrdU ( Fig. 5c,f ), indicating that SVZ NPCs and virus-infected striatal cells generated new neurons at distinct locations. 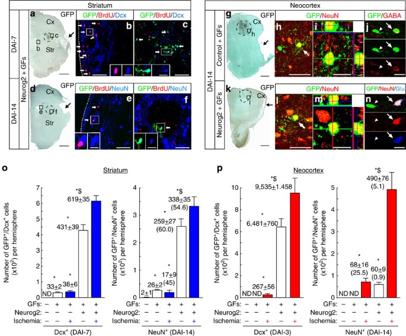Figure 5: Neurogenesis in the ischaemic brain. (a–n) BrdU- and GFP-labelled neurons in the adult rat striatum (a–f) and neocortex (g–n). Circles and boxes ina,d,g,kindicate the location of virus-infected cells and the areas shown in fluorescence images, respectively. Dashed lines inbandeindicate the ventricular wall.bandeshow BrdU-labelled neurons near the LV, whereascandfshow GFP-labelled neurons detected around virus-infected regions in the striatum.handjshow GFP+/NeuN+and GFP+/GABA+cells, respectively, in the neocortex that received control viruses, whereaslandnshow GFP+/NeuN+and GFP+/NeuN+/Glu+cells, respectively, detected in Neurog2 virus-infected animals.iandmshow orthogonal views of z-stack confocal images of neurons indicated by arrows inhandl, respectively. (o,p) Estimated numbers of GFP+/Dcx+cells at DAI-3 (neocortex) and DAI-7 (striatum) (o), and GFP+/NeuN+cells at DAI-14 (both regions) (p) under various manipulation conditions (mean±s.d.,n=3–4 animals). The data regarding non-ischaemic animals are adopted fromFig. 3d,e. The numbers in parentheses show the percentage of GFP+/NeuN+cells at DAI-14 compared with GFP+/Dcx+cells at earlier time points. *P<0.01 compared with control viruses in Student’st-test; $P<0.01 compared with non-ischaemic animals treated with GFs and Neurog2 in Student’st-test. ND, not detected. Scale bar,a,d,g,k, 2 mm;b,c,e,f,h,l, 50 μm; and insets inb,c,e,f,i,j,m,n, 20 μm. Figure 5: Neurogenesis in the ischaemic brain. ( a – n ) BrdU- and GFP-labelled neurons in the adult rat striatum ( a – f ) and neocortex ( g – n ). Circles and boxes in a , d , g , k indicate the location of virus-infected cells and the areas shown in fluorescence images, respectively. Dashed lines in b and e indicate the ventricular wall. b and e show BrdU-labelled neurons near the LV, whereas c and f show GFP-labelled neurons detected around virus-infected regions in the striatum. h and j show GFP + /NeuN + and GFP + /GABA + cells, respectively, in the neocortex that received control viruses, whereas l and n show GFP + /NeuN + and GFP + /NeuN + /Glu + cells, respectively, detected in Neurog2 virus-infected animals. i and m show orthogonal views of z-stack confocal images of neurons indicated by arrows in h and l , respectively. ( o , p ) Estimated numbers of GFP + /Dcx + cells at DAI-3 (neocortex) and DAI-7 (striatum) ( o ), and GFP + /NeuN + cells at DAI-14 (both regions) ( p ) under various manipulation conditions (mean±s.d., n =3–4 animals). The data regarding non-ischaemic animals are adopted from Fig. 3d,e . The numbers in parentheses show the percentage of GFP + /NeuN + cells at DAI-14 compared with GFP + /Dcx + cells at earlier time points. * P <0.01 compared with control viruses in Student’s t -test; $ P <0.01 compared with non-ischaemic animals treated with GFs and Neurog2 in Student’s t -test. ND, not detected. Scale bar, a , d , g , k , 2 mm; b , c , e , f , h , l , 50 μm; and insets in b , c , e , f , i , j , m , n , 20 μm. Full size image New neurons were barely detectable in control virus-infected, non-ischaemic neocortex ( Fig. 5p ). We found, however, a small number of GFP + cells expressing Dcx and NeuN in the ischaemic cortex ( Fig. 5h–i ). Co-treatment with Neurog2 viruses and GFs induced a larger number of GFP + cells to express Dcx (1.5-fold) and NeuN (8.2-fold; Fig. 5p ). Moreover, more Dcx + cells seemed to proceed to NeuN + neurons between DAI-7 and DAI-14 after ischaemia (5.1 versus 0.9%), suggesting that ischaemia augments both the production and subsequent maturation/survival of new neurons. Interestingly, about half of GFP + /NeuN + cells in control virus-infected neocortex were GABA + (12/23 cells) but none of them were Glu + (0/28 cells) or GluR2/3 + (0/34 cells; Fig. 5i ). By contrast, all GFP + /NeuN + cells examined were Glu + (27/27 cells) and GluR2/3 + (15/15 cells) in Neurog2 virus-treated animals ( Fig. 5n ). Thus, Neurog2 seemed to promote differentiation of glutamatergic neurons in the adult neocortex as in embryos [32] , [33] . GFs increase cells capable of forming neurospheres Recent studies have shown that skin fibroblasts can be reprogrammed to become neurons [18] , [19] , [20] , [21] , [22] , [23] , [24] , [25] , [26] as well as NPCs [35] , [36] , [37] , [38] . The aforementioned data also show that some GFP-labelled neurons originate from cells that divide in situ . Such dividing cells could be either NPCs or other cell types. To test the former possibility, we asked whether cells labelled with GFP viruses in vivo are capable of forming neurospheres, a hallmark of NPCs in vitro . We administered GFs and control viruses to adult rats and subsequently isolated small pieces of tissue around the injection sites at DAI-3. In the presence of FGF2 and EGF, 0.61±0.26% of SVZ-derived cells formed neurospheres, whereas such cells was rare in the neocortex and striatum of uninjured brains (0.03±0.02% and 0.09±0.03%, respectively; Fig. 6a–j and Table 1 ). The content of sphere-forming cells in the corpus callosum, which has been reported to contain NPC-like cells [39] , was also extremely low (0.005±0.001%; Fig. 6j ). However, tissues that received stab wound and GFs yielded many more neurospheres than control as reported in previous studies [28] , [29] , [40] ( Fig. 6c–e , Table 1 ). Most of these GFP + spheres were composed entirely of GFP + cells (355/362 striatum-derived spheres and 89/90 cortex-derived spheres examined; Fig. 6a,b ), and conversely, the rest of the spheres contained few, if any, GFP + cells, demonstrating the clonal expansion of GFP + neurospheres. After passage, these primary spheres formed secondary spheres composed of cells incorporating BrdU, indicating that they were proliferating in vitro ( Fig. 6f–h ). Moreover, the frequency of cells forming secondary spheres within primary spheres was comparable between the three regions ( Fig. 6j ). When these secondary neurospheres were induced to differentiate in monolayer, the percentage of TuJ1 + neurons among total cells was also similar in the three cultures ( Fig. 6i,m ). The ratio of GFAP + astrocytes, however, was about twofold higher in the SVZ-derived culture, and the cortical culture contained a higher percentage of O4 + oligodendrocytes compared with the other two regions ( Fig. 6k–m ). These results support the idea that stab wound and GFs promotes the generation of NPC-like cells in vivo . 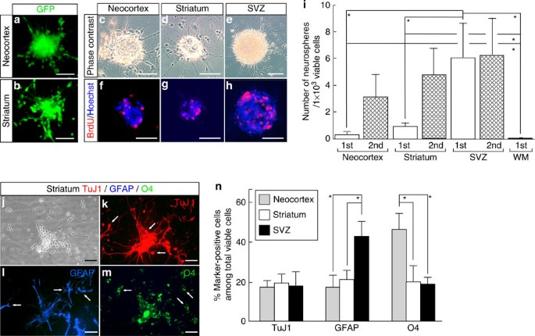Figure 6: Neurosphere-forming cells induced by stab wound and GFs in the adult rat neocortex and striatum. (a,b) GFP+neurospheres formedin vitroby cells exposed to GFs and GFP virusesin vivo. (c–h) Phase-contrast images (c–e) and staining for BrdU (f–h, red) of growing secondary neurospheres. Cell nuclei were stained with Hoechst 33258 (blue). (i) Frequencies of neurosphere-forming cells 14 days after tissue isolation (primary spheres, indicated as 1st) and 14 days after the first passage (secondary spheres, indicated as 2nd; mean±s.d.,n=10). *P<0.01 in Student’st-test. (j–m) Differentiation of a secondary neurosphere derived from the striatum. The cells (phase-contrast image inj) were stained for TuJ1 (k, red), GFAP (l, blue) and O4 (m, green). (n) Percentages of TuJ1+, GFAP+and O4+cells among total cells in culture of secondary neurospheres (mean±s.d.,n=4). *P<0.01 compared with SVZ-derived cells in Student’st-test. Scale bar,a,b,d–i,k, 50 μm. Figure 6: Neurosphere-forming cells induced by stab wound and GFs in the adult rat neocortex and striatum. ( a , b ) GFP + neurospheres formed in vitro by cells exposed to GFs and GFP viruses in vivo . ( c – h ) Phase-contrast images ( c – e ) and staining for BrdU ( f – h , red) of growing secondary neurospheres. Cell nuclei were stained with Hoechst 33258 (blue). ( i ) Frequencies of neurosphere-forming cells 14 days after tissue isolation (primary spheres, indicated as 1st) and 14 days after the first passage (secondary spheres, indicated as 2 nd ; mean±s.d., n =10). * P <0.01 in Student’s t -test. ( j – m ) Differentiation of a secondary neurosphere derived from the striatum. The cells (phase-contrast image in j ) were stained for TuJ1 ( k , red), GFAP (l, blue) and O4 ( m , green). ( n ) Percentages of TuJ1 + , GFAP + and O4 + cells among total cells in culture of secondary neurospheres (mean±s.d., n =4). * P <0.01 compared with SVZ-derived cells in Student’s t -test. Scale bar, a , b , d – i , k , 50 μm. Full size image Table 1 Neurosphere formation by virus-infected cells in vitro. Full size table Distinct gene expression profiles of NPC-like cells We next isolated similar NPC-like cells from the adult mouse brain and characterized their properties by microarray-based gene expression profiling. Among 41,170 probes covering the mouse genome, we identified 3,781 probes representing 3,003 genes that gave more than a five-fold higher hybridization signal with one or more of the adult neurosphere-forming cells compared with the whole brain ( Fig. 7a ). Clustering analyses of three independent samples demonstrated a reproducible gene expression profile of cells derived from each region ( Fig. 7b ). Among these genes, 1,558 genes were common between cells from all three regions, whereas 435 and 58 genes were uniquely enriched in neocortical and striatal cells, respectively ( Fig. 7a ). 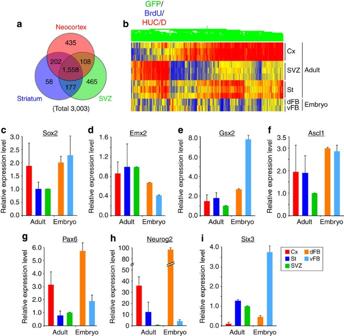Figure 7: Differential gene expression profiles of neurosphere-forming cells derived from distinct regions of the adult mouse brain. (a) Venn diagram showing the number of genes commonly and differentially expressed in neurospheres derived from the SVZ, neocortex and striatum. Among 3,003 genes that were selected as those that gave more than a five-fold higher hybridization signal with one or more of the adult neurosphere samples compared with the whole brain of adult mice. (b) Heat-map view of cluster analysis of 716 probe sets (637 genes) that showed more than a five-fold difference in the expression level between cortical and SVZ cells (three stripes represent three independent cultures). Neurospheres from the dorsal and ventral forebrains (dFB and vFB, respectively) of E14.5 embryos were used for comparison. (c–i) Quantitative RT-PCR analyses of the expression of TF mRNAs. The levels are normalized using glyceraldehyde-3-phosphate dehydrogenase as internal control and data are expressed as values relative to the SVZ-derived cells (designated as 1.0; mean±s.d.,n=3). dFB, dorsal embryonic forebrain culture; vFB, ventral embryonic forebrain culture. Figure 7: Differential gene expression profiles of neurosphere-forming cells derived from distinct regions of the adult mouse brain. ( a ) Venn diagram showing the number of genes commonly and differentially expressed in neurospheres derived from the SVZ, neocortex and striatum. Among 3,003 genes that were selected as those that gave more than a five-fold higher hybridization signal with one or more of the adult neurosphere samples compared with the whole brain of adult mice. ( b ) Heat-map view of cluster analysis of 716 probe sets (637 genes) that showed more than a five-fold difference in the expression level between cortical and SVZ cells (three stripes represent three independent cultures). Neurospheres from the dorsal and ventral forebrains (dFB and vFB, respectively) of E14.5 embryos were used for comparison. ( c – i ) Quantitative RT-PCR analyses of the expression of TF mRNAs. The levels are normalized using glyceraldehyde-3-phosphate dehydrogenase as internal control and data are expressed as values relative to the SVZ-derived cells (designated as 1.0; mean±s.d., n =3). dFB, dorsal embryonic forebrain culture; vFB, ventral embryonic forebrain culture. Full size image Many genes commonly expressed in embryonic and adult NPCs encode TFs [41] . We thus focused our initial analysis on this class of genes. Neurospheres isolated from the dorsal and ventral forebrains of E14.5 embryos (dFB and vFB, respectively) were included for comparison. Some TFs were expressed at similar levels (less than twofold difference) across adult cells, which included Sox2, Emx2, Gsx2 and Ascl1 ( Fig. 7c–f ). Sox2 is ubiquitously expressed in undifferentiated progenitors, whereas Emx2 is expressed in a forebrain-specific manner during development [39] . Their expression thus reflects their common properties as NPCs with a forebrain identity. Although the expression of Gsx2 and Ascl1 is mostly confined in the vFB in embryos [42] , we detected similar expression levels of these TFs across the adult and embryonic cells. By contrast, Pax6 and Neurog2 were expressed in higher levels in neocortical cells than SVZ and striatal cells, whereas Six3 was expressed in an opposite manner ( Fig. 7g–i ). These patterns mirror the difference between the embryonic dFB and vFB, the primordia of the adult neocortex and striatum, respectively [42] . We confirmed the expression of some of these TFs at the protein level by immunostaining ( Supplementary Fig. S5 ). These results demonstrate that NPC-like cells induced in the adult neocortex and striatum exhibit distinct molecular profiles in vitro . Although we examined whether GFP-labelled cells express any of these TFs in stab-wounded animals in situ , we could not find such cells. It could be that such cells exist only transiently or in small number, or manifest unique molecular phenotypes after expansion in vitro . Thus, the biological relevance of each of these genes in the context of in vivo reprogramming remains to be further investigated. Recent studies have demonstrated that a variety of non-neuronal cells can be reprogrammed to become neurons and NPCs in vitro [18] , [19] , [20] , [21] , [22] , [23] , [24] , [25] , [26] , [35] , [36] , [37] , [38] , [43] , [44] , [45] , [46] . Other studies have also shown that fully differentiated cells acquire the properties of tissue-specific stem cells in vivo under certain circumstances [4] , [5] , [6] , [7] . In line with these emerging findings, we found that exposure to GFs and overexpression of the neurogenic TF Neurog2, in combination of stab wound, can induce new neurons in the adult neocortex and striatum where neuronal turnover is otherwise absent or extremely rare [12] , [13] . Stab wound or ischaemia alone did not induce such neurogenesis at a significant level, indicating that GFs and Neurog2 exert unique actions to reprogramme non-neuronal cells. In vivo treatment with GFs and Neurog2 also increased the frequency of cells that were capable of forming neurospheres in vitro , suggesting that the production of neurons occurs, at least in part, through the generation of NPC-like cells. Interestingly, such NPC-like cells derived from different regions exhibited distinct molecular profiles in vitro . Thus, reprogrammed cells in the adult brain seem to inherit distinct properties of the cells of their origin. Whether such differences are attributable to their intrinsic properties or the influence of their environment remains to be examined. The retrovirus used in this study infected many different cell types in vivo , yet only a small fraction of infected cells were reprogrammed to become neurons. Thus, the identity of cells that retain a competency to become neurons in response to GFs and Neurog2 is currently unknown. Various cell types, including astrocytes and pericytes in the brain, have been shown to be reprogrammable to neurons and NPCs in vitro [18] , [19] , [20] , [21] , [22] , [23] , [24] , [25] , [26] , [43] , [44] , [45] , [46] . Recent studies also suggest that certain glial cells such as reactive astrocytes and NG2 + glial progenitors exhibit a capacity for neurogenesis in vitro [28] , [29] , [40] and in vivo [47] , [48] . Thus, these glial cells may serve as the source of new neurons. In fact, a recent study has demonstrated the generation of new neurons by direct conversion of astrocytes in the striatum in vivo [10] . These cells, however, comprised a minor fraction of total virus-infected cells in our study. Thus, given the reported low efficiency of neuronal reprogramming of each of these cell types in vitro , it could be that GF/Neurog2-induced neurons originate from multiple non-neuronal cells rather than one specific cell type. Alternatively, the adult neocortex and striatum may contain cells that intrinsically retain the properties of NPCs but remain dormant in the intact brain. In this scenario, the action of GFs and Neurog2 is to mobilize them to differentiate into neurons. In fact, previous studies have reported the occurrence of such cells outside the known neurogenic niches [28] , [29] , [40] , [49] , [50] . An important finding in this study is that the in vivo environment affects many aspects of neuronal reprogramming in vivo . In the striatum, GFs or Neurog2 alone induced a small but significant number of new neurons after stab wound, and their combination further stimulated local neurogenesis. In the neocortex, however, Neurog2 alone induced a large number of immature neurons, but only a small number of mature neurons remained at later stages. A previous study has also shown that overexpression of Pax6 and a dominant-negative form of Olig2 induces immature but not mature neurons in the adult neocortex [8] . Thus, neuronal reprogramming seems to be more restricted in the neocortex than in the striatum. Interestingly, both the production and subsequent maturation of new neurons were enhanced after focal ischaemia in the neocortex. Thus, stab wound and ischaemia modulate local neurogenesis in different manners. Our data have also demonstrated that the in vivo environment strongly influences the molecular phenotypes of newly generated neurons in vivo . What mechanisms underlie these differences is currently unknown. It could be attributable to differences in the intrinsic properties of cells or environmental regulations, or both. Differential inflammatory and immune responses or expression of distinct GFs, cytokines and morphogens could underlie the region- and injury-specific regulation of neurogenesis [16] , [51] . If reprogrammed neurons are to be utilized for the brain repair, it is crucial to understand the nature of these environmental signals and their mechanisms of action. Whether new neurons generated in injured brains contribute to functional recovery also needs to be further investigated. Although our preliminary studies did not detect significant impact of neuronal reprogramming in vivo on behavioural recovery after stab wound or ischaemic injury, it could be because of the relatively small number of new neurons induced by the method employed in this study. Yet, it is encouraging that recent studies have shown that exogenous NPC-derived or reprogrammed neurons, when transplanted in a large number, can be integrated into the existing circuitry and contribute to certain function, demonstrating that the adult mammalian brain is receptive to new neurons [18] , [19] , [20] , [21] , [22] , [23] , [24] , [25] , [26] , [43] , [44] , [45] , [46] , [52] , [53] , [54] , [55] . Further understanding of the environmental impact on neuronal reprogramming in vivo may lead to the development of new strategies to augment the latent regenerative potential of the adult brain. Animals Adult male Sprague–Dawley rats (10–12 weeks of age, 300–360 g) were used in all in vivo experiments. Adult male CD1 mice (10–12 weeks of age, 30–40 g) were used for gene expression profiling of neurospheres. All animal procedures were performed according to the guidelines of the Institutional Animal Care and Use Committee and the National Institute of Health. Retrovirus infection and other in vivo manipulations High-titer solutions (2 × 10 8 colony-forming unit per ml) of recombinant retroviruses pMXIG and its derivatives expressing Neurog2, Pax6 and Ascl1 (refs 9 , 14 , 31 ) were prepared with artificial cerebrospinal fluid (124 mM NaCl, 5 mM KCl, 1.3 mM MgCl 2 , 2 mM CaCl 2 , 26 mM NaHCO 3 and 10 mM D -glucose, with the pH adjusted to 7.2 using aeration with 95% O 2 –5% CO 2 ) containing rat serum albumin (1 mg ml −1 , Sigma-Aldrich). In some experiments, the virus solution was supplemented with FGF2 (0.9 μg ml −1 ; Peprotech) and EGF (0.9 μg ml −1 ; Roche). The virus solution was delivered into the brain through an infusion cannula with an external guide cannula (Plastic One) at a flow rate of 1 μl min −1 with an automated injection pump (BASi) attached to a stereotaxic injection device (Narishige, Tokyo, Japan) [44] . For injection into the striatum, the cannula was placed 0 mm anterior and 3.0 mm lateral from bregma and the cannula tip was placed 4.0 mm deep from the skull surface. This stereotaxic coordinate targeted the middle of the dorsal aspect of the striatum of adult rats [56] . Injection into the frontal area of the neocortex was performed with the cannula placed 2.5 mm anterior and 2.0 mm lateral from bregma and the depth was 2.0 mm. After injection, the cannula was left for additional 10 min before removing. BrdU labelling To label proliferating cells in the brain, BrdU (150 mg kg −1 of body weight, Sigma-Aldrich) dissolved in 0.9% sterile saline was injected intraperitoneally in two different paradigms. In the pre-labelling paradigm, BrdU was administered to animals twice a day for 3 consecutive days, and subsequently viruses were injected into the brain 24 h after the last BrdU injection. In the post-labelling experiments, the first administration of BrdU was performed 2 h after virus injection, and subsequently repeated every 12 h for 3 days. Retrograde axonal tracing One microlitre of artificial cerebrospinal fluid containing 3% (w/v) FluoroGold (FG) was injected into the globus pallidus ipsilateral to the virus injection site [57] . The stereotaxic coordinates were 2.3 mm posterior and 4.0 mm lateral to bregma and the cannula depth was 6.8 mm 5 (ref. 5 ). FG was injected 84 days after virus infection and animals were killed at day 91. Serial sections of the brain were examined to confirm that bulk labelling was confined to the globus pallidus without significant passive diffusion into adjacent regions. Focal cortical ischaemia Rats were anaesthetized with isoflurane (2.0% (v/v)) and maintained at the lateral position with mechanical ventilation (1% isoflurane in a mixture of 30% O 2 and 70% N 2 O). The blood gas conditions were kept at the constant levels (PO 2 , 120±10 mm Hg; PCO 2 , 35±3 mm Hg) and the rectal and temporal muscle temperatures were maintained at 37.5±0.2 and 37.0±0.1 °C, respectively, throughout the surgery. The distal branch of the middle cerebral artery was exposed at its proximal trunk through the subtemporal approach, thermo-coagulated with a bipolar coagulator (MIZUHO Co., Ltd., Tokyo, Japan) and severed with a microscissor at the position just distal to the lenticulostriate branch. This occlusion causes localized damage in the dorsolateral neocortex, whereas the rest of the neocortex and other brain regions remain mostly intact [34] . After surgery, animals were maintained on a heating blanket to prevent hypothermia until they began spontaneous movement, and were subsequently returned to their home cages and individually housed. For subsequent 3 days, animals were inspected daily to ensure that they had access to food and water. Histological analysis For quantification of GFP- and BrdU-labelled cells, every 10 sections among serial coronal sections of the entire striatum (−0.3 to +1.6 mm from bregma, ~95 sections) or the anterior part of the neocortex (+3.2 to +4.7 mm from bregma, ~75 sections) were subjected to immunostaining. Among all animals examined, the maximum dispersion of GFP + cells was observed in an area of ~2.0 mm 3 in volume (anteroposterior, 1.0 mm; dorsoventral, 1.0 mm; and mediolateral, 2.0 mm) in both the striatum and neocortex; but in most cases, they were confined to a smaller area (<1.0 mm 3 ). GFP + cells (50–500) were detected per section depending on its distance from the injection site. The total number of GFP + cells and the percentage of cells double stained for specific markers were estimated in each manipulated animal, and the results are expressed as mean±s.d. of the data obtained from three to four independent animals. To validate the co-staining of multiple markers in single cells, samples were examined by confocal Z-sectioning at an interval of 1.0 mm using LSM-510 (Carl Zeiss). Only cells that appeared to retain the intact soma and nuclei within a given section, which was judged according to the staining pattern of GFP and BrdU, were counted. At least 100 or more double-labelled cells were observed using confocal microscope in representative sections from animals treated under different conditions. Quantification of the number and density of BrdU-labelled cells in the SVZ and parenchyma was performed using four representative coronal sections from each animal in which a cluster of GFP + cells were detected around the injection site. The SVZ was defined as the 100-μm-wide region lining the LV. Immunostaining Animals were euthanized with CO 2 and fixed using intracardiac perfusion with 4% (w/v) paraformaldehyde (Acros Organics). Brains were collected and post-fixed with paraformaldehyde for an additional 12 h. Subsequently, the samples were cryoprotected with sucrose and embedded into an optimal cutting temperature compound (Sakura Finetek, USA). Twenty micrometre-thick sagittal or coronal sections were serially collected on slide glasses and subjected to immunostaining [9] , [14] . When staining was visualized with a colorimetric substrate for peroxidase (Pierce), sections were counterstained with methylgreen (Sigma-Aldrich). Images were captured using the CCD camera Pixera Pro 600ES attached to the microscope BX-50 (Olympus). Images after staining with secondary antibodies conjugated with fluorescence probes were obtained with the Axiophoto2 (Carl Zeiss) equipped with the CCD camera C5810 (Hamamatsu Photonics) or with LSM-510 (Carl Zeiss). The antibodies used for immunostaining are listed in Supplementary Table S2 . Neurosphere culture One millimetre-thick serial coronal slices of brains were prepared using the rodent brain matrix (ASI Instruments). The striatum and dorsofrontal cortex were microdissected under the binocular microscope SV-11 (Carl Zeiss). Rat brain tissues were isolated from the slices encompassing ~+3.5 to +2.0 mm from bregma for the neocortex and −0.5 to +1.5 mm for the striatum using the optic chiasm as an anatomical landmark [5] . For mouse brains, slices encompassing ~+1.4 to +0.0 mm from bregma were used [58] . In both cases, incisions were placed at least 0.5 mm away from the visible borders of the LV and corpus callosum to avoid contaminations of the adjacent white matter and periventricular tissue. A stripe of tissue lining the LV (~100 μm thick) was collected as a specimen containing the SVZ. For gene expression profiling studies, the dFB and vFB, which contain the embryonic primordia of the neocortex and striatum, respectively, were isolated from mouse embryos at embryonic day E14.5 (refs 59 , 60 ). Dissociated single cells were seeded at a density of 1 × 10 4 cells per ml in a growth medium (1:1 mixture of Dulbecco’s modified Eagle’s medium and F-12 medium (Invitrogen) supplemented with B-27 and N2 supplements (Invitrogen), 20 ng ml −1 FGF2, 20 ng ml −1 EGF, 20 ng ml −1 platelet-derived GF (Roche), 2 μg ml −1 heparin sulphate (molecular mass of 3,000; Sigma-Aldrich), 1 mg ml −1 bovine serum albumin (Sigma-Aldrich) and 100 μM 2-mercaptoethanol (Sigma-Aldrich) [9] , [14] , [31] . Culture dishes were coated with 20 mg ml −1 poly (2-hydroxy-ethyl methacrylate) (Sigma-Aldrich) to prevent cell attachment. At day 14 in vitro (DIV-14), the number of neurospheres with a diameter over 100 mm was counted. Subsequently, these primary neurospheres were subjected to serial passages under the same conditions. BrdU (0.5 μM; Sigma-Aldrich) was added to the culture of secondary neurospheres for 3 days between DIV-14 and DIV-17 to detect dividing cells in neurospheres. In some experiments, brains that received retrovirus infection in vivo (see below) were subjected to neurosphere culture. The site of virus injection in coronal slices was identified under the microscope and small piece of tissue around the injection site was removed. A portion of the sample was subjected to immunostaining for GFP and the number of GFP + cells among total viable cells was quantified. The rest of the sample was subjected to neurosphere culture as described above. To induce differentiation, primary or secondary neurospheres were seeded onto poly- D -lysine (100 μg ml −1 ; Sigma-Aldrich)-coated eight-well chambers (Nalge Nunc), either as cell aggregates (~20 spheres per well) or at a density of 2 × 10 4 cells per well after dissociation. The resultant cells were further cultured in a growth medium without GFs. The cells were subjected to immunostaining for TuJ1, GFAP and O4 at DAI-10. Immunoreactive cells were visualized with secondary antibodies conjugated with Alexa Fluor dyes (1:200; Invitrogen). To count cell numbers, cell nuclei were stained with 1 μg ml −1 Hoechst 33258 (Invitrogen). Gene expression profiling Secondary neurospheres derived from different brain regions were subjected to gene expression profiling studies using microarrays. Three sets of adult mouse brain-derived cells were obtained from independent culture experiments. Freshly isolated tissues and neurospheres derived from the dFB and vFB of E14.5 mice were used for comparison. RNeasy mini kit (QIAGEN) was used for isolation and purification of total RNAs. The concentration of RNA was measured using RNA Assay Nanoprep Chip 6000 and Bioanalyzer (Agilent). To compare the expression profiles across the samples, Affymetrix GeneChip Mouse Genome 430 2.0 Array Platform (total 41,170 probes) was used and the data were analysed using Silicon Genetics GeneSpring Software GX7.3.1. To identify genes enriched in NPCs and NPC-like cells, we used a data set of the whole brain of adult mice that were obtained using the same microarray platform and made available by the Gene Expression Omnibus Project on the website of the National Center for Biotechnology Information (accession number GDS592: http://www.ncbi.nlm.nih.gov/geo/gds/gds_browse.cgi?gds=592 ). The data were normalized to median settings across the entire probe set and samples, and transcript levels fivefold or higher than those in the adult brain were taken as significant enrichment. The relative mRNA expression levels of selected genes were quantified by quantitative reverse transcriptase PCR analysis using Opticon DNA Engine (BIO-RAD). Glyceraldehyde-3-phosphate dehydrogenase was used as an internal control and statistical significance was evaluated by two-tailed unpaired t -test. The primers used are listed in Supplementary Table S3 . Accession codes: Microarray data have been deposited in Gene Expression Omnibus under the Accession Code GSE49194 . How to cite this article: Grande, A. et al. Environmental impact on direct neuronal reprogramming in vivo in the adult brain. Nat. Commun. 4:2373 doi: 10.1038/ncomms3373 (2013).